Predicting oculomotor behaviour from correlated populations of posterior parietal neurons Oculomotor function critically depends on how signals representing saccade direction and eye position are combined across neurons in the lateral intraparietal (LIP) area of the posterior parietal cortex. Here we show that populations of parietal neurons exhibit correlated variability, and that using these interneuronal correlations yields oculomotor predictions that are more accurate and also less uncertain. The structure of LIP population responses is therefore essential for reliable read-out of oculomotor behaviour. The cortical signals that support sensory representations and motor commands are arguably carried by neuronal populations [1] , [2] , [3] . The correlated variability between the responses of neurons in an ensemble is a fundamental property of the population response [4] , [5] , [6] . In computational and systems neuroscience, cortical signals are often studied by predicting sensory inputs and behaviours from ensembles of neurons. Many reports have focused on the accuracy of these predictions, particularly the impact of interneuronal correlations [1] , [2] , [4] , [7] , [8] , [9] , [10] , [11] . However, little is known about the uncertainty of these predictions. For instance, a correct estimate may be more valuable to an organism faced with making a decision if this estimate has low uncertainty. If the same estimate has high uncertainty, the organism may choose to delay the decision until it can obtain an estimate with lower uncertainty. Furthermore, the relation between the prediction accuracy and uncertainty remains an open question, for example, is an accurate prediction also less uncertain? To address this issue, we examined how oculomotor behaviours could be predicted from the responses of neuronal populations in the sensorimotor cortex. We used a Bayesian framework and studied the posterior distribution: the probability of an oculomotor behaviour given a population response [12] . The behavioural estimate corresponding to a given neuronal population response is commonly represented by the mean of the posterior distribution (alternatively, the estimate can also be represented by the location of the maximum or the median). 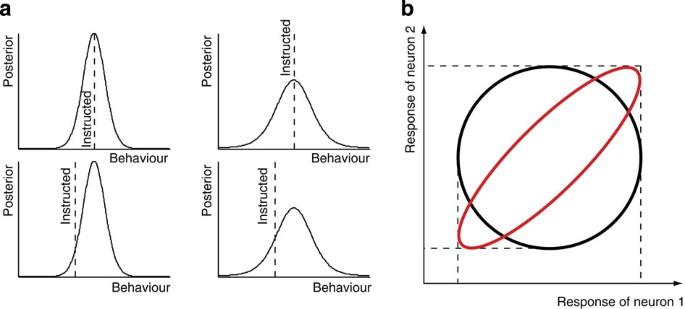Figure 1: Illustration of prediction metrics and the impact of interneuronal correlations. (a) Difference between prediction accuracy and uncertainty. (b) Impact of interneuronal correlations on the shape of the neuronal response distribution of two neurons. Figure 1a shows four different posterior distributions yielding correct (mean of distribution aligned with instructed behaviour, first row) and incorrect estimates (mean misaligned with instructed behaviour, second row). The posterior distributions in the first and second columns also differ by their width. The posteriors in the left column are sharper than in the right column. This geometrical property is captured by the variance of the posterior distribution. We define the uncertainty of the behavioural estimate inferred from a given population response as the variance of the posterior distribution. Because a posterior is a probability density function (positive function that sums to 1), a lower variance is also accompanied by a peak of higher amplitude. Thus, an estimate that has low uncertainty is derived from a posterior that is sharply peaked and has high amplitude. By nature, the mean and the variance of the posterior are independent ( Fig. 1a ). The prediction uncertainty is a metric quantifying the width of the peak, if any, of the posterior distribution, while the prediction error measures the location of this peak. For instance, if the neuronal correlates of an oculomotor behaviour yield a posterior distribution with a sharp peak at the correct location, the estimate will be accurate and will have a low uncertainty (top, left). If this peak is not very pronounced (top, right), the prediction, although still correct, will have high uncertainty, thus reflecting the fact that the prediction will be very sensitive to ‘noise’ because the peak of an almost flat distribution can wander widely. The uncertainty is thus a complementary metric to the prediction accuracy (for example, the difference between the predicted estimate and the instructed one) that allows gauging the reliability of an estimate. Figure 1: Illustration of prediction metrics and the impact of interneuronal correlations. ( a ) Difference between prediction accuracy and uncertainty. ( b ) Impact of interneuronal correlations on the shape of the neuronal response distribution of two neurons. Full size image Predictions from neuronal populations depend on the interneuronal correlations between pairs of neurons [1] , [2] , [3] , [4] , [5] , [6] . On the basis of the geometry of the neuronal response distributions, it has been suggested that positive interneuronal correlations could potentially help and negative correlations hinder prediction accuracy [1] . We hypothesize that interneuronal correlations can only decrease the prediction uncertainty ( Fig. 1b ). By keeping the marginal projections (the variance that is) constant, the effect of adding neuronal correlations to an uncorrelated response distribution (black circle) creates a distribution (red ellipse) that can only be sharper, and potentially yield an estimate with a lower uncertainty. Therefore, interneuronal correlations can impact prediction accuracy and uncertainty differently. It is however still unclear how the geometry of the neuronal response distributions relates to the prediction accuracy through the computation of the posterior distribution. The lateral intraparietal (LIP) area is a cortical sensorimotor area known to represent saccades and eye position [13] , [14] , [15] , [16] , [17] . It is a central node in the processing of sensorimotor function. Surprisingly, LIP has only been recently studied at the level of neuronal populations [18] . However, it is still unknown whether LIP neurons exhibit correlated variability and how these interneuronal correlations affect the prediction of oculomotor behaviours. We determined the accuracy and uncertainty of sensorimotor predictions based on the responses from populations of LIP neurons of two nonhuman primates and investigated the effect of the correlated variability between neurons on these predictions. We found that eye position and saccade direction predictions that incorporate the correlated variability between neurons are more accurate and less uncertain. We recorded 51 populations composed on average of ~7 neurons, for a total of 343 neurons. The monkeys made instructed delayed memory saccades between the nodes of a Cartesian grid by starting the saccade on a 3 × 3 grid spaced by 8° and moving their gaze to one of the 8 neighbouring nodes ( Fig. 2a ). This task allowed us to independently study the neuronal correlates of saccade direction and the (initial) eye position during the six task epochs ( Fig. 2b ). 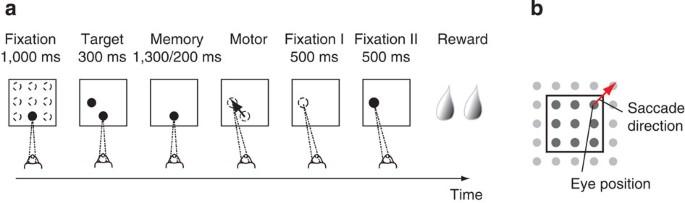Figure 2: Delayed memory saccade task on a grid. (a) Schematic showing the six task epochs. (b) Instructed saccade directions and eye positions on a Cartesian grid. Figure 2: Delayed memory saccade task on a grid. ( a ) Schematic showing the six task epochs. ( b ) Instructed saccade directions and eye positions on a Cartesian grid. Full size image We present empirical evidence that the responses of LIP neurons have correlated variability in the awake nonhuman primate. We obtained a total of 1,044 spike count correlations (see Methods) for each of the six task epochs ( Fig. 3a ). These interneuronal correlations only slightly varied across task epochs, suggesting that the different cognitive states of the animal had a limited impact on the mean correlated variability of LIP neurons. These correlations were surprisingly high, as also illustrated by their average strength across epochs ( Fig. 3b ). The magnitude of interneuronal correlations in LIP was comparable to previous findings [5] in visual cortex (for example, in V1, V2, V4 and MT) and higher than expected from reports in motor areas (for example, M1, SMA, FEF) and in cognitive areas (for example, perirhinal and prefrontal). This finding highlights the place of LIP as a sensorimotor area that is a node between the visual input and motor output. The dependency between signal and spike count correlations was weak ( Fig. 3c ), similarly to previous reports in visual cortex [19] . Similarly, the relation between interneuronal correlations and the geometric mean of the spike count [20] was faint ( Fig. 3d ). Taken together, both findings suggest that the tuning difference between two LIP neurons is only slightly informative about their correlated variability. 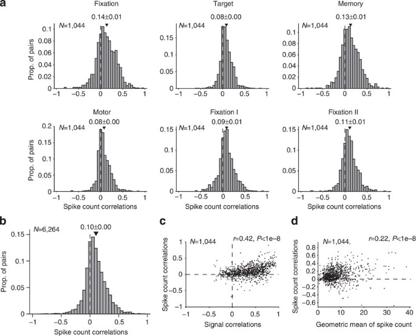Figure 3: Spike count correlations between pairs of neurons. (a) Distribution of spike count correlations across all pairs of simultaneously recorded neurons for each epoch of the task. (b) Distribution of spike count correlations across all pairs of simultaneously recorded neurons and across task epochs. (c) Relation between spike count and signal correlations. (d) Relation between spike count correlations and the geometric mean of the spike count. Figure 3: Spike count correlations between pairs of neurons. ( a ) Distribution of spike count correlations across all pairs of simultaneously recorded neurons for each epoch of the task. ( b ) Distribution of spike count correlations across all pairs of simultaneously recorded neurons and across task epochs. ( c ) Relation between spike count and signal correlations. ( d ) Relation between spike count correlations and the geometric mean of the spike count. Full size image We then asked how interneuronal correlations affected the prediction of saccade direction and eye position from the spike count across each task epoch. For this, we computed the probability of an oculomotor behaviour given a population response (the posterior distribution). To explicitly represent interneuronal correlations, we assumed that the spike count statistics were described by a truncated multivariate Gaussian distribution. The covariance matrix was assessed for each behaviour separately, thus leading to a reduced number of trials available to its estimation, and ultimately to an approximation that would poorly generalize (overfit). To resolve this, we used a Tikhonov regularization to shrink the covariance matrix towards a lower-dimensional representation [21] . This allowed us to derive two types of decoders. The Gaussian decoder GD used interneuronal correlations, and as such had access to the full covariance matrix of the spike counts across trials for each behavioural condition. Its correlation-blind variant, the CB-GD, only used the diagonal terms of the covariance matrix (the variance of the spike counts), and as such is often referred to as a diagonal decoder [1] . The comparison between the two decoders allowed us to assess the impact of interneuronal correlations on predicting sensorimotor functions. The behavioural estimate corresponding to a given neuronal population response was the mean of the posterior distribution, and the prediction accuracy was the proportion of estimates falling within 11.25° of veridical for saccade direction and within 2° of veridical for eye position across all trials for each population and task epoch (a quarter of the task discretization for each behavioural variable). The accuracy of the predictions of the GD was on average 8.1±0.9% and 5.9±0.9% higher than for the CB-GD for saccade direction and eye position, respectively. These results show that oculomotor behaviour can be more accurately predicted when the decoder uses interneuronal correlations, similar to previous reports [4] , [22] . Notably, our populations were relatively small, and as such there were only a small number of interneuronal correlations available to the decoder to increase the prediction accuracy (the off-diagonal terms of the covariance matrix). To put these results in perspective, we evaluated the separability of artificial neuronal population responses with different magnitudes of interneuronal correlations (see Methods). We found that neuronal responses with correlations similar to the empirically derived ones ( r ~0.1) could be separated 6.89±0.23% (mean and s.d.) better than without interneuronal corrections ( r =0). This result supports our empirical findings and also strengthens the relationship between prediction accuracy and neuronal population response. Furthermore, this numerical exercise allowed us to assess whether the increase in decoding accuracy was merely a consequence of the decoder using one more parameter, namely interneuronal correlations. For this, we evaluated the separability of neuronal population responses for a low magnitude of interneuronal correlations ( r =0.01). We found that under these circumstances the neuronal responses could still be better separated than without correlations (0.69±0.02%, mean and s.d. ), albeit less well than above where r ~0.1. This finding shows that the empirical increase in prediction accuracy we found when comparing the GD with the CB-GD was not due to simply using an additional parameter for decoding, it was the magnitude of these correlations that was responsible for the better performance of the GD. We then compared the CB-GD with another inference scheme, the Poisson independent decoder PID, where the posterior is computed assuming a Poisson response distribution and neuronal independence [4] , [8] , [9] , [10] , [18] . The CB-GD yielded a prediction accuracy that was 10.2±1.0% and 10.9±1.2% superior to the PID for saccade direction and eye position, respectively. This finding illustrates that the CB-GD was able to better represent the empirical structure of the data than the PID because it used a larger number of parameters (mean and variance of spike counts versus mean only) to better fit the neuronal data. Our results show that predictions based on a decoder that uses interneuronal correlations are more accurate. It is however unclear whether these predictions are accompanied by a higher certainty because prediction error (location of mean of the posterior) and uncertainty (width of the peak of the posterior) are independent. To address this issue, we examined the joint and marginal distributions of the prediction error (the difference between the instructed and the predicted behaviour) and prediction uncertainty for saccade direction and eye position across neuronal populations, task epochs and trials ( Fig. 4a,b ). The joint two-dimensional (2D) distributions of the prediction error and uncertainty for the GD showed that correct predictions were associated with the lowest uncertainty: the joint distributions peaked when the prediction error and uncertainty were both nil (deep red regions). This was more readily visible by looking at the peaks of the marginal distributions (the red curves corresponding to the GD). The joint distributions also reflected the discrete nature of the behaviours sampled by our task, for example, the ‘forbidden’ half discs showing that some error and uncertainty combinations did not occur. Finally, the joint distributions encoded the periodicity of the represented variable. The saccade direction is a periodic variable with a periodicity of 360°. Its joint prediction distribution therefore wrapped around the abscissa and exhibited continuity between 180° and −180°. The eye position, however, was not periodic, and its joint distribution did not wrap around at 16° and −16°. This finding suggests that different cortical representations (continuous and non-continuous) are used to infer saccade directions and eye positions. 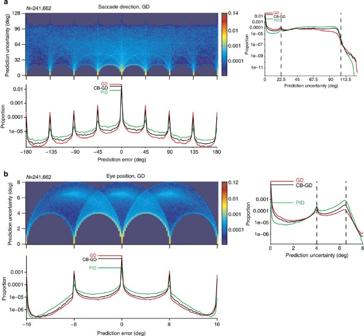Figure 4: Joint and marginal distributions of the prediction error and prediction uncertainty. (a) Distributions for the saccade direction across populations, epochs and trials. (b) Distributions for the eye position across populations, epochs and trials. Figure 4: Joint and marginal distributions of the prediction error and prediction uncertainty. ( a ) Distributions for the saccade direction across populations, epochs and trials. ( b ) Distributions for the eye position across populations, epochs and trials. Full size image The marginal 1D distributions of the prediction error corroborated our previous findings. The GD yielded the most accurate predictions for the saccade direction and eye position: the peaks of the distributions, indicated by the horizontal lines, were highest for the GD (red), lower for the CB-GD (black) and lowest for the PID (green). This finding shows again that the more complicated quadratic decoding scheme of the GD and CB-GD outperformed the simple linear PID, and that interneuronal correlations increased the prediction accuracy of oculomotor behaviour from populations of intraparietal neurons. We also found that the three decoders, despite their different assumptions, had an increased number of estimates close to the behaviours cued by the task, thus reflecting a neuronal representation that yielded an almost discretized set of behavioural predictions. In accord with the above finding about the periodicity of the representation, our findings show that the neuronal representations follow the nature of the oculomotor behaviours imposed by the task, here the periodicity of the saccade direction. The marginal 1D distributions of the prediction uncertainty showed that the GD yielded the highest proportion of lowest uncertainty for the saccade direction and eye position, followed by the CB-GD and finally the PID. The quadratic decoding schemes thus yielded estimates that were less uncertain than the linear decoder, and using interneuronal correlations decreased the uncertainty of the estimates. The uncertainty distributions also had a similar shape for the three decoders. The locations peaks in these distributions were however less straightforward to predict. When predicting saccade direction ( Fig. 4a ), the first peak of uncertainty was at 0 and corresponded to a posterior with no uncertainty: one saccade direction had a probability of 1 and all the other ones had a probability of 0 (Dirac-like posterior). The second peak occurred for an uncertainty close to 22.5° (dotted line) corresponding to a posterior where two saccade directions were equiprobable (that is, with a probability of 0.5 each), and all the other saccade directions had a probability of 0. Furthermore, we found that most of the encountered posteriors were not close to being flat (where every saccade direction has an equal probability of 1/8), which would correspond to an uncertainty close to the dotted line at 105.5°. We found similar results when predicting the eye position ( Fig. 4b ), except that the peaks for the uncertainty were at 0°, 4° and 6.53° (1-valued, 2-valued and uniform posteriors, respectively). While the peaks of the prediction error distributions informed about the discretization of the task, the peaks of the uncertainty distributions yielded a measure of the shape of the posterior distributions used to predict oculomotor behaviours from populations of LIP neurons. Prediction error and uncertainty are both properties of the neuronal data brought to light by a specific decoding framework, in our case Bayesian inference. These metrics quantify how oculomotor function is encoded by neuronal ensembles. We showed that eye position and saccade direction predictions that incorporated the correlated variability between neurons were more accurate and less uncertain. Our results show that interneuronal correlations in area LIP of the posterior parietal cortex play an important role in sharpening the representation of saccade direction and eye position during oculomotor behaviour. Neuronal population recordings We previously described the recording procedure [18] . Briefly, we recorded populations of LIP neurons in two adult male rhesus monkeys ( Macaca mulatta ) using a 5-channel microdrive with movable electrodes. Single units were sorted online using a dual-window discriminator based on the shape of the waveform. We used magnetic resonance imaging scans as guides for the location of LIP. At the beginning of each recording session, we verified that each electrode tip was located in LIP by obtaining vigorous visual, motor planning and motor activity during a centre-out delayed memory saccade task. Each animal was recorded in a different hemisphere. We acquired a different population of simultaneously recorded neurons for each session. All procedures were in accordance with the guidelines of the Caltech Institutional Animal Care and Use Committee and the National Institute of Health Guide for the Care and Use of Laboratory Animals. Delayed memory saccade task on a grid The animals performed delayed memory saccades on a Cartesian grid whose nodes were spaced by 8° ( Fig. 1 ). The animals maintained fixation for 1,000 ms at one randomly chosen location on the 3 × 3 grid. Next a target was flashed for 300 ms in one location randomly chosen from the eight neighbouring locations, and the animals were required to maintain fixation during this epoch. The animals had to remember the target location for 1,300±200 ms (drawn from a uniform distribution). On extinction of the fixation, they made a saccade to the remembered target location in complete darkness, thus acquiring a postsaccade fixation on a 5 × 5 grid. They maintained fixation there for 500 ms (fixation I) in the absence of visual input. A fixation light was subsequently turned on at the target location for another 500 ms, possibly triggering a small corrective saccade. On completion of this second fixation (fixation II), the stimulus was removed and the animals were rewarded with water drops. We only considered correct trials. The animals completed ~11 random blocks, for a total of ~11 × ((3 × 3) × 8)=792 saccades. The eye position was tracked by an infrared camera, and the signal was sampled at 2 kHz. All behavioural variables were instructed and monitored in real time [18] . Spike count correlations For each pair of simultaneously recorded neurons, we determined the spike count correlation in each task epoch similarly to a previously described method [19] . Briefly, we computed for both neurons the Z -score of the spike count of the trials corresponding to a given saccade direction and eye position. We then combined these values across the nine presaccade eye positions and eight saccade directions (for a total of 72 oculomotor behaviours), removed the outliers ( Z -score >3) and finally computed the Pearson correlation coefficient between both neurons. Neuronal data The neuronal data were the spike count for each neuron in each task epoch. Our task design exhaustively sampled eight saccade directions and nine presaccade eye positions, for a total of 72 oculomotor behaviours. Each of these behaviours was executed on average 11 times. One caveat of reliably assessing interneuronal correlations is to gather a large number of trials for each behaviour because correlations are a second-order statistic. Because presaccade eye position and saccade direction were two independent variables in our task, we studied them separately by creating two data sets. The saccade direction data set combined for each saccade direction the responses across all eye positions, thus yielding on average 99 trials for each of the eight saccade directions. The eye position data set combined the responses across all saccade directions for each eye position and gave on average 88 trials for each of the nine eye positions. Simply combining the responses would increase the variability for each behaviour because LIP neurons exhibit a joint encoding of saccade direction and eye position, a property termed gain fields [13] , [14] . We took this into account and scaled each of the responses with their average gain field before combining them. The saccade direction and the eye position data sets were thus two different representations of the same underlying data. We inferred saccade direction using the saccade direction data set and eye position using the eye position data set. Inferring eye position and saccade direction We modelled decoding using the posterior distribution p ( b| r ): the probability to obtain a behaviour b given a neuronal population response r . By Bayes’ theorem [12] , the posterior is proportional to the product of the likelihood function p ( r |b ) and the prior p ( b ): The prior function is simply the probability of occurrence of a behaviour and was thus entirely defined by the task (no error trials). The likelihood function captures the encoding process: it is the probability to obtain a population response r given a behaviour b , evaluated across behaviours. We assumed that the encoding process was described by a multivariate Gaussian distribution, yielding the following log-likelihood function: where N is the number of neurons in a population, μ ( b ) the average response across trials for the behaviour b and Σ( b ) the covariance matrix across trials for the behaviour b . The log-likelihood function is quadratic in the neuronal response. The virtue of this parametric representation is that it explicitly represents interneuronal correlations, as opposed to implicit representations [4] . As such, the impact of correlations on decoding can simply be assessed by removing the non-diagonal terms of the covariance matrix, effectively using only the variance of the neuronal response. The Gaussian model is a parametric approximation of the neuronal response distribution that belongs to the exponential family [6] , [7] , which also includes the Poisson independent approximation [4] , [8] , [9] , [10] . Although neuronal responses are positive integers, the Gaussian distribution can have negative tails. In that case, the Gaussian distribution is not normalized for positive values. We corrected this by normalizing the Gaussian distribution as follows: with To compute the correction factor, we assumed the covariance matrix to be diagonal to reduce the complexity of the numerical integration. Because Σ( b ) is computed for each behaviour, its evaluation is less robust than the one of the spike count correlation where trials across behaviours were combined (see above). Thus, to ensure a good generalization ability of the estimate for Σ( b ), we chose to regularize it with the identity matrix within a convex hull [21] and imposed one regularizer across all behaviours for each population: The cost function was the proportion of veridical estimates derived from the maximum of the posterior. The cost function was fivefold cross-validated [23] . We maximized the cost function using an exhaustive search to avoid local maxima. We used this technique to derive the GD by regularizing the full covariance matrix, and also its correlation-blind variant CB-GD by separately regularizing a diagonal covariance matrix. Finally, we evaluated the posterior function using a leave-one-out cross-validation scheme to ensure good generalization and avoid overfitting [23] . To compute the prediction accuracy, we considered the mean, or first moment, of the posterior distribution, effectively assuming a quadratic loss function [24] . This so-called Bayesian estimate was then used to determine the prediction error and the proportion of estimates close to veridical. The uncertainty of this estimate was the variance, or second moment, of the posterior distribution. Separability of neuronal population responses We modelled the separability of neuronal population responses for varying magnitudes of the interneuronal correlations. For this, we generated artificial populations of correlated neurons that had similar physiological properties as our empirical neuronal samples. We simulated population responses to a preferred and to an anti-preferred saccade direction using circular Gaussian functions. We used a previously established model [11] to create correlated neurons for each saccade direction. Briefly, we multiplied normally distributed random numbers with the matrix square root of the correlation matrix and scaled the results using the mean and variance of the spike counts. We then examined how well the correlated population responses corresponding to the preferred and anti-preferred directions could be separated. We used a Fisher linear discriminant analysis that finds a direction that yields the best separation between the projected neuronal responses corresponding to the two saccade directions [23] . This direction maximizes the Rayleigh quotient of the within-class and the between-class scatter matrices, and it is derived from the sum of the within-class scatter matrices corresponding to the two saccade directions. We finally computed the Fisher score by projecting on this direction the difference between the correlated neuronal population data corresponding to each direction. The Fisher score allowed us to assess how well the responses corresponding to two stimuli could be separated: a large Fisher score was indicative of responses that differed strongly, whereas a small Fisher score indicated responses that could not well be distinguished. We reported the relative increase in Fisher scores derived from correlated neuronal populations with respect to uncorrelated ones. How to cite this article: Graf, A. B. A. and Anderson, R. A. Predicting oculomotor behaviour from correlated populations of posterior parietal neurons. Nat. Commun. 6:6024 doi: 10.1038/ncomms7024 (2015).